A peptide probe for targeted brown adipose tissue imaging The presence of brown adipose tissue responsible for thermogenic energy dissipation has been revealed in adult humans and has high clinical importance. Owing to limitations of current methods for brown adipose tissue detection, analysing the abundance and localization of brown adipose tissue in the body has remained challenging. Here we screen a combinatorial peptide library in mice and characterize a peptide (with the sequence CPATAERPC) that selectively binds to the vascular endothelium of brown adipose tissue, but not of intraperitoneal white adipose tissue. We show that in addition to brown adipose tissue, this peptide probe also recognizes the vasculature of brown adipose tissue-like depots of subcutaneous white adipose tissue. Our results indicate that the CPATAERPC peptide localizes to brown adipose tissue even in the absence of sympathetic nervous system stimulation. Finally, we demonstrate that this probe can be used to identify brown adipose tissue depots in mice by whole-body near-infrared fluorescence imaging. The metabolic state of the body depends on the balance between the two adipose tissue depots: white adipose tissue (WAT) and brown adipose tissue (BAT) [1] , [2] . Although WAT stores excess energy in the form of neutral triglycerides, BAT dissipates energy in the form of heat. Differentiated cells of BAT, brown adipocytes, have comparatively small lipid droplets, abundant mitochondria, and specifically express molecules such as uncoupling protein 1 (UCP1) to direct the respiratory chain toward fast substrate oxidation with a low rate of ATP production [3] . The adaptive thermogenesis function of BAT has been established predominantly through studies in rodents that contain substantial BAT depots in adulthood. For some adipose tissue depots, a conversion between WAT and BAT has been revealed, which depends on the delicate balance between caloric intake and sympathetic nervous system stimuli through cold temperature and other beta-3 adrenergic signals. In humans, BAT is clearly present and functional in newborns, whereas adults had been thought to lack BAT. Recently, a number of groups reported the presence of functional BAT in adults through the use of positron emission tomography (PET) based on the uptake of fluorine-18 deoxyglucose (FDG) by metabolically active BAT [4] , [5] , [6] , [7] , [8] . As this method is limited by its dependence on fluctuating metabolic activity [9] of BAT, as well as false-positive signals from other metabolically active tissues [10] , new approaches for BAT identification would be highly beneficial. In this study, we aimed at developing a non-invasive method for identification of BAT in the mouse model. Our previous studies have demonstrated that in vivo screening of phage-displayed combinatorial peptide libraries in animals and end-of-life patients enables identification of probes recognizing vascular surface molecules expressed in an organ-selective manner [11] , [12] , [13] , [14] , [15] . Such peptide probes have been applied for direction of imaging agents and therapeutics to tissues of interest, including WAT, in animal models [16] , [17] , [18] , [19] . We hypothesized that the vascular proteome of BAT may also be distinct from that of other organs and that differentially expressed surface molecules may enable identification of probes selective for BAT. Based on these considerations, we set out to use the mouse model to screen for BAT-homing peptides, with the end-point goal of testing them in imaging applications aimed at detecting BAT within surrounding tissues ( Fig. 1a ). 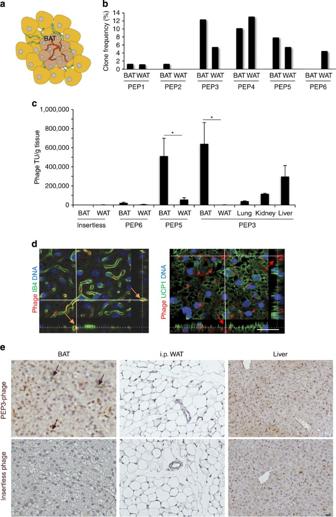Figure 1: A screen for BAT-homing peptides. (a) The hypothesis: endothelium of BAT expresses specific surface receptors. (b) Comparison of recovery frequency for phage clones displaying peptides (PEP1 through PEP6) from BAT and WAT at round 3 of combinatorial library selection in mouse BAT. (c) Validation of BAT homing for selected phage-displayed peptides compared to peptide-free phage (insertless) through administration of 109transforming units (TU) into mice. After 1 h of circulation, PEP3-phage displays superior selectivity of accumulation in BAT but not in control organs. Error bars: s.e.m. *P<0.05 (Student’st-test);n=3 (different phage titration dilutions). (d) Anti-phage immunofluorescence (red) upon injection into a mouse revealed in BAT sections. Confocal Z-stack projections of median series demonstrate luminal localization of PEP3-phage in vessels of BAT revealed by IB4 labelling (green, left), but not to adipocytes expressing UCP1 (green, right). (e) Anti-phage immunohistochemistry (brown) showing that PEP3-phage homes to vessels of BAT (arrows), but not of i.p. WAT. Mouse injected with insertless phage has no BAT or WAT signal, and liver trapping of phage is comparable to trapping of PEP3-phage. Hematoxylin counterstaining: blue. Nuclei are blue. For all cases, scale bar, 20 μm. Figure 1: A screen for BAT-homing peptides. ( a ) The hypothesis: endothelium of BAT expresses specific surface receptors. ( b ) Comparison of recovery frequency for phage clones displaying peptides (PEP1 through PEP6) from BAT and WAT at round 3 of combinatorial library selection in mouse BAT. ( c ) Validation of BAT homing for selected phage-displayed peptides compared to peptide-free phage (insertless) through administration of 10 9 transforming units (TU) into mice. After 1 h of circulation, PEP3-phage displays superior selectivity of accumulation in BAT but not in control organs. Error bars: s.e.m. * P <0.05 (Student’s t -test); n =3 (different phage titration dilutions). ( d ) Anti-phage immunofluorescence (red) upon injection into a mouse revealed in BAT sections. Confocal Z-stack projections of median series demonstrate luminal localization of PEP3-phage in vessels of BAT revealed by IB4 labelling (green, left), but not to adipocytes expressing UCP1 (green, right). ( e ) Anti-phage immunohistochemistry (brown) showing that PEP3-phage homes to vessels of BAT (arrows), but not of i.p. WAT. Mouse injected with insertless phage has no BAT or WAT signal, and liver trapping of phage is comparable to trapping of PEP3-phage. Hematoxylin counterstaining: blue. Nuclei are blue. For all cases, scale bar, 20 μm. Full size image Here we report the results of the screen for BAT-homing peptides. We characterize a peptide termed PEP3 that targets the endothelium of BAT and of metabolically active subcutaneous (sc) WAT. By conjugating PEP3 with a near-infrared (NIR) fluorophore, we test the capacity of this probe to localize BAT by whole-body imaging. We demonstrate that PEP3 identifies mouse BAT even under conditions of sympathetic nervous system inhibition and low UCP1 expression. Screen for BAT-homing peptides To isolate peptides that home to adult BAT in vivo , we used a mixture of cyclic CX 7 C and CX 8 C (C: disulfide-bonded cysteines; X: any amino acid) peptide libraries [12] . This mixed library with a combined diversity of ~10 11 was subjected to a selection in Sv129 mice that accumulate well defined BAT depots [20] . Low temperature (6 °C) acclimation was used as a condition leading to activation of BAT metabolic activity [10] , [21] , [22] . In each round, an intravenously (i.v.) injected library phage suspension was allowed to circulate in a cold-acclimated animal for 1 h, and phage particles were recovered from interscapular BAT and from intraperitoneal (i.p.) WAT as a control. The BAT-recovered phage pool was used for the subsequent selection in C57BL/6 mice housed at room temperature that display comparatively low level of BAT activation [20] , which was done to avoid isolation of peptides with background-selective properties. After three rounds of such in vivo biopanning, sequencing of DNA coding for peptide inserts revealed the selection of six peptide sequences repeatedly recovered from BAT or WAT with frequency above 1%. These peptides were termed PEP1 through PEP6 and had the following sequences: CLNGLGRGRC (PEP1); CWSIGNGSLC (PEP2); CPATAERPC (PEP3); CNFGHVGGC (PEP4); CLATSEVVC (PEP5) and CKEMSALKLC (PEP6). PEP3 binds to endothelium of brown and beige adipose tissue Phage displaying PEP3 showed the best BAT enrichment: it constituted 12.2% of the BAT-recovered clones and was recovered from WAT at lower frequency ( Fig. 1b ). Administration of individual peptide-displaying phage clones into cold-acclimated mice and quantification of phage particles in tissues demonstrated PEP3-phage and PEP5-phage accumulation in BAT being significantly higher than for control insertless phage and PEP6-phage ( Fig. 1c ). PEP3-phage displayed the highest specificity for BAT compared with i.p. WAT, lungs and kidneys ( Fig. 1c ). As reported previously [13] , [19] , we observed nonspecific trapping of phage in liver ( Fig. 1c ); which was comparable for all phage clones. Confocal immunofluorescence analysis of BAT from mice injected with PEP3-phage demonstrated its luminal localization in microvessels of BAT stained with isolectin B4 (IB4) labelling the endothelium [23] , while no phage co-localization was observed for adipocytes expressing UCP1 ( Fig. 1d ). Immunohistochemical analysis of tissues from mice injected with individual phage-displayed peptide clones confirmed PEP3-phage localization to the lumen of capillaries in interscapular BAT. We did not detect PEP3-phage in i.p. WAT, while the amount of PEP3-phage nonspecifically trapped in the liver was comparable to that observed for peptide-free phage ( Fig. 1e ). To determine whether cell populations other than the endothelium are targeted by PEP3, we analysed cells recovered from BAT of cold-acclimated mice 1 h after PEP3-phage injection by flow cytometry. Based on the cell surface marker combinations previously established for cell populations in adipose tissue [12] , [24] , [25] , [26] , we used fluorescence-activated cell sorting (FACS) to separate BAT cells into CD31+CD34dimCD45- endothelial cells, CD31-CD34brightCD45- stromal cells, CD31-CD34-CD45- preadipocytes, and CD45+ leukocytes. Quantification of phage particles recovered with each population demonstrated that PEP3 binds to the endothelium but not to other BAT cell populations analysed ( Fig. 2a ). Analysis of adherent stromal/vascular fraction demonstrated that 44±9% of CD31+ cells contained phage particles ( Fig. 2b,c ). To test whether PEP3 is capable of targeting BAT endothelium outside of the phage context, we i.v. injected cold-acclimated mice with chemically synthesized PEP3 that was labelled with the Cy3 fluorophore. Analysis of Z-stack projections in BAT recovered 1 h after peptide administration by confocal immunofluorescence indicated that PEP3-Cy3 was associated with BAT vasculature and not with adipocytes expressing UCP1 ( Fig. 2d ). We also tested if PEP3 binds to the endothelium in a tissue culture setting. The stromal/vascular cells isolated from mouse BAT were subjected to brown adipogenesis induction in adherent culture as described [27] . Upon lipid droplet formation in differentiated adipocytes, we incubated the cells in adherent culture with PEP3-Cy3. After washing off unbound peptide, we fixed the cells and subjected them to anti-CD31 or anti-UCP1 immunofluorescence. Expression of CD31 in cell networks indicated the retention of endothelial cells, while UCP1 expression confirmed brown adipocyte differentiation ( Fig. 2e ). Although PEP3 binding to vascular networks was not uniform, suggesting peptide selectivity for a subset of endothelial cells, we did observe peptide co-localization with CD31-positive structures ( Fig. 2e ). According to quantification, 40±7% of CD31+ cells were bound by the peptide ( Fig. 2f ). These data suggest that PEP3 may have selectivity for a subtype of endothelial cells. There was a general lack of PEP3 co-localization with UCP1-positive adipocytes ( Fig. 2e ), confirming peptide specificity for the endothelium. 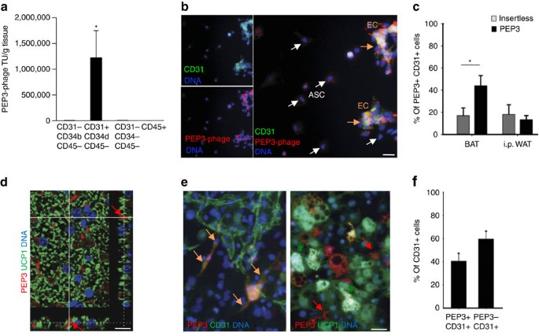Figure 2: PEP3 targets BAT endothelium. (a) 1 h after PEP3-phage injection into a mouse, BAT cells were separated by FACS and recovery of TU (per gram of tissue ±s.e.m.;n=2 different phage titration dilutions) was graphed for CD31+CD34dimCD45- endothelial cells, CD31-CD34brightCD45- stromal cells, CD31-CD34-CD45- preadipocytes, and CD45+ leukocytes. (b) BAT-derived cells from mice injected with PEP3-phage or insertless phage were analysed in adherent culture using anti-CD31 and anti-phage antibodies. Immunofluorescence reveals CD31+ endothelial cells (green) containing PEP3-phage (red speckles) in contrast to CD31− cells (ASC) showing only background autofluorescence. (c) Frequency of CD31+ cells from the mouse analysed in (b) stained positive with anti-phage antibodies (mean±s.e.m.,n=14). (d) Immunofluorescence analysis of BAT from a mouse i.v.-injected with 60 nmol of PEP3-Cy3 (red) demonstrating peptide accumulation in the vessels (arrow) but not in adipocytes expressing UCP1 (green). Confocal Z-stack projections demonstrate lack of green and red signal co-localization. (e) The stromal/vascular cells of mouse BAT subjected to brown adipogenesis induction in adherent culture were incubated with PEP3-Cy3 (5 μg ml−1) and then fixed and subjected to anti-CD31 or anti-UCP1 immunofluorescence (green). Yellow arrows: bound PEP3 co-localized with endothelial networks (left). Red arrows: lack of bound PEP3 co-localization with UCP1-expressing adipocytes (green, right). (f) Adherent BAT-derived cells were incubated with PEP3-Cy3 (5 μg ml−1). Plotted is the frequency of CD31+ cells bound with PEP3 (mean±s.e.m.,n=12). Nuclei are blue. All scale bars, 20 μm. *P<0.05 (Student’st-test). Figure 2: PEP3 targets BAT endothelium. ( a ) 1 h after PEP3-phage injection into a mouse, BAT cells were separated by FACS and recovery of TU (per gram of tissue ±s.e.m. ; n =2 different phage titration dilutions) was graphed for CD31+CD34dimCD45- endothelial cells, CD31-CD34brightCD45- stromal cells, CD31-CD34-CD45- preadipocytes, and CD45+ leukocytes. ( b ) BAT-derived cells from mice injected with PEP3-phage or insertless phage were analysed in adherent culture using anti-CD31 and anti-phage antibodies. Immunofluorescence reveals CD31+ endothelial cells (green) containing PEP3-phage (red speckles) in contrast to CD31− cells (ASC) showing only background autofluorescence. ( c ) Frequency of CD31+ cells from the mouse analysed in ( b ) stained positive with anti-phage antibodies (mean±s.e.m., n =14). ( d ) Immunofluorescence analysis of BAT from a mouse i.v.-injected with 60 nmol of PEP3-Cy3 (red) demonstrating peptide accumulation in the vessels (arrow) but not in adipocytes expressing UCP1 (green). Confocal Z-stack projections demonstrate lack of green and red signal co-localization. ( e ) The stromal/vascular cells of mouse BAT subjected to brown adipogenesis induction in adherent culture were incubated with PEP3-Cy3 (5 μg ml −1 ) and then fixed and subjected to anti-CD31 or anti-UCP1 immunofluorescence (green). Yellow arrows: bound PEP3 co-localized with endothelial networks (left). Red arrows: lack of bound PEP3 co-localization with UCP1-expressing adipocytes (green, right). ( f ) Adherent BAT-derived cells were incubated with PEP3-Cy3 (5 μg ml −1 ). Plotted is the frequency of CD31+ cells bound with PEP3 (mean±s.e.m., n =12). Nuclei are blue. All scale bars, 20 μm. * P <0.05 (Student’s t -test). Full size image To investigate time-dependence of PEP3 retention in BAT, we performed comparative analysis of tissues from cold-acclimated mice 1 and 4 h after PEP3-Cy3 i.v. injection. By co-staining tissue sections with fluorophore-conjugated IB4 labelling the endothelium [23] , we observed clear intravascular/luminal peptide localization at both time points, although upon prolonged peptide circulation the signal intensity was diminished ( Fig. 3a ). Peptide fluorescence was undetectable in i.p. WAT of the same mice ( Fig. 3a ). Confocal fluorescence analysis did not reveal peptide penetration into non-vascular cells of BAT. To determine whether PEP3 homing to BAT relies on its metabolic activity, we administered PEP3-Cy3 into warm-acclimated mice. Confocal co-localization with IB4 revealed PEP3-Cy3 in BAT vasculature 1 h after i.v.-injection ( Fig. 3b ). A control peptide CSWKYWFGEC (WAT7) that homes to WAT [12] was not detected in BAT ( Fig. 3c ). PEP3 biodistribution was assessed through the analysis of control tissues ( Fig. 3d ). PEP3 was occasionally observed in sc WAT, but not detectable in i.p. WAT, skeletal muscle and lungs. As expected, PEP3 was detectable in kidneys, the site of peptide clearance. We also detected signal in liver; however, it was predominantly non-endothelial and comparable to that observed for the control peptide CSWKYWFGEC ( Fig. 3c ). This nonspecific signal could be explained by trapping of free Cy3 fluorophore, produced from peptide proteolysis. 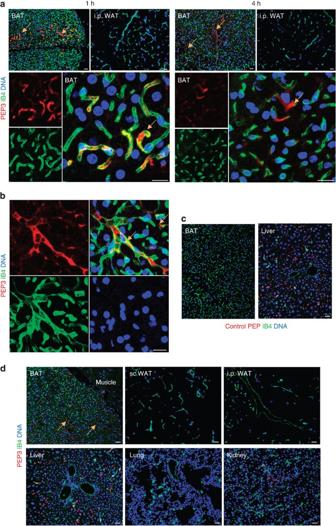Figure 3: PEP3 localizes to BAT vasculature in cold- and warm-acclimated mice. Confocal fluorescence analysis of tissue sections from after i.v.-injection of 60 nmol of indicated Cy3-conjugated peptide. Endothelium is labelled with IB4 (green). Arrows indicate PEP3 localization in the vasculature of BAT. (a) PEP3 in BAT, but not i.p. WAT, of cold-acclimated mice 1 h and 4 h post-injection. High-magnification images (lower panels) demonstrate that peptide localization is exclusively intravascular/luminal (yellow). (b) PEP3 in BAT vasculature of warm-acclimated mice 1 h post-injection. (c) Control WAT-homing peptide WAT7 (ref.12) detected in liver (non-endothelial) but not in BAT 1 h post-injection into warm-acclimated mice. (d) PEP3 detected in BAT, and occasionally in sc WAT, but not in i.p. WAT, muscle or lungs, 1 h post-injection into warm-acclimated mice. Occasional kidney and liver PEP3 trapping (non-endothelial) is comparable to that of the Control peptide. Nuclei are blue. For all cases, scale bar, 20 μm. Figure 3: PEP3 localizes to BAT vasculature in cold- and warm-acclimated mice. Confocal fluorescence analysis of tissue sections from after i.v.-injection of 60 nmol of indicated Cy3-conjugated peptide. Endothelium is labelled with IB4 (green). Arrows indicate PEP3 localization in the vasculature of BAT. ( a ) PEP3 in BAT, but not i.p. WAT, of cold-acclimated mice 1 h and 4 h post-injection. High-magnification images (lower panels) demonstrate that peptide localization is exclusively intravascular/luminal (yellow). ( b ) PEP3 in BAT vasculature of warm-acclimated mice 1 h post-injection. ( c ) Control WAT-homing peptide WAT7 (ref. 12 ) detected in liver (non-endothelial) but not in BAT 1 h post-injection into warm-acclimated mice. ( d ) PEP3 detected in BAT, and occasionally in sc WAT, but not in i.p. WAT, muscle or lungs, 1 h post-injection into warm-acclimated mice. Occasional kidney and liver PEP3 trapping (non-endothelial) is comparable to that of the Control peptide. Nuclei are blue. For all cases, scale bar, 20 μm. Full size image Comparative immunofluorescence analysis of tissue sections from warm- and cold-acclimated mice confirmed UCP1 induction by cold temperature in BAT. PEP3-Cy3 localized to BAT vasculature despite the reduction in UCP1 expression level ( Fig. 4a,b ). As reported previously [21] , [28] , sc WAT upon cold acclimation contained vast areas of ‘beige’ (‘brite’) adipocytes expressing UCP1, which were also present, albeit less abundant, in warm-acclimated mice ( Fig. 4a ). We observed PEP3-Cy3 homing to vessels associated with the UCP1-expressing adipocytes in sc WAT of both cold- and warm-acclimated animals ( Fig. 4a ), indicating that PEP3 receptor is also expressed by vasculature of metabolically active beige adipose tissue. 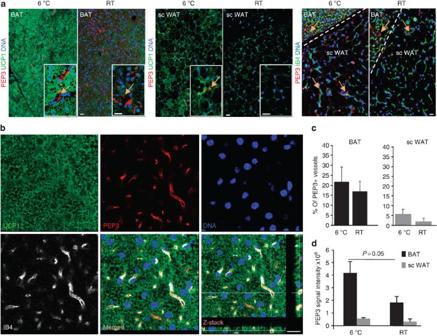Figure 4: PEP3 localizes to vasculature of BAT and metabolically active sc WAT. (a) Confocal immunofluorescence analysis of tissue sections from cold (6 °C) or warm (RT) -acclimated mice 1 h after i.v.-injection of PEP3-Cy3. Anti-UCP1 (green) immunofluorescence demonstrates UCP1 induction by cold in both BAT and WAT. Insets (high-magnification) show PEP3 vascular homing (arrow), to UCP1-expressing areas. IB4 co-localization shows PEP3-Cy3 presence in interscapular sc WAT adjacent to BAT. (b) Three-color confocal immunofluorescence analysis of BAT sections from a cold-acclimated mouse 1 h after i.v. injection of PEP3-Cy3 showing co-localization of PEP3 (red) with an endothelial marker IB4 (white), but not with brown adipocyte-expressed UCP1 (green). Z-stack projections confirm co-localization of IB4 and PEP3. (c) Tissue sections (n=5) from cold- and warm-acclimated mice injected with PEP3-Cy3 were analysed and the percentage of microvessels associated with PEP3-Cy3 signal (mean± s.e.m.) was plotted. (d) Cumulative PEP3-Cy3 pixel intensity (mean± s.e.m.) in sections (n=4) of indicated tissues was measured by Amira 5.4 (VSG) software. Nuclei are blue. For all cases, scale bar, 20 μm. Figure 4: PEP3 localizes to vasculature of BAT and metabolically active sc WAT. ( a ) Confocal immunofluorescence analysis of tissue sections from cold (6 °C) or warm (RT) -acclimated mice 1 h after i.v.-injection of PEP3-Cy3. Anti-UCP1 (green) immunofluorescence demonstrates UCP1 induction by cold in both BAT and WAT. Insets (high-magnification) show PEP3 vascular homing (arrow), to UCP1-expressing areas. IB4 co-localization shows PEP3-Cy3 presence in interscapular sc WAT adjacent to BAT. ( b ) Three-color confocal immunofluorescence analysis of BAT sections from a cold-acclimated mouse 1 h after i.v. injection of PEP3-Cy3 showing co-localization of PEP3 (red) with an endothelial marker IB4 (white), but not with brown adipocyte-expressed UCP1 (green). Z-stack projections confirm co-localization of IB4 and PEP3. ( c ) Tissue sections ( n =5) from cold- and warm-acclimated mice injected with PEP3-Cy3 were analysed and the percentage of microvessels associated with PEP3-Cy3 signal (mean± s.e.m.) was plotted. ( d ) Cumulative PEP3-Cy3 pixel intensity (mean± s.e.m.) in sections ( n =4) of indicated tissues was measured by Amira 5.4 (VSG) software. Nuclei are blue. For all cases, scale bar, 20 μm. Full size image PEP3 signal in BAT vasculature appeared patchy, indicating that its binding to the endothelium is not homogenous at the dose used. To quantify this, we determined the percentage of microvessels associated with PEP3-Cy3 using tissue sections. Comparison of BAT from cold- and warm-acclimated mice showed that the percentage of microvessels associated with PEP3-Cy3 was not significantly different ( Fig. 4c ). However, peptide signal intensity in BAT vessels appeared higher for cold-acclimated than for warm-acclimated mice ( Fig. 3a,d ). Quantification demonstrated that cumulative PEP3 signal intensity was elevated ( P =0.05, Student’s t -test) in BAT of cold-conditioned mice ( Fig. 4d ). This result indicates that the probe homing to BAT is increased by its metabolic activity and suggests that PEP3 receptor, constitutively expressed in BAT at a basal level, is upregulated by sympathetic stimuli. PEP3 test in NIR-imaging applications Next we tested whether peptides can be used as probes for whole-body BAT imaging. Based on our expertise, a fluorophore that emits in the NIR range was selected to give the advantage of comparatively high tissue penetration and low background [29] , [30] . IRDye800 was conjugated with PEP3 via amide linkage to a lysine residue inserted at the N-terminus and analysed by HPLC ( Fig. 5a ); as controls, we used IRDye800-labelled WAT-homing peptide CKGGRAKDC [18] and PEP1, which showed no preference for BAT over i.p. WAT ( Fig. 1b ). In a dose escalation experiment, Sv129 mice pre-housed at 6 °C were i.v. injected with 2, 5, 10, 30 and 60 nanomoles (nmol) of PEP3-IRDye800 and whole-body NIR-fluorescence imaging was performed. To identify tissues containing the peptide, we exposed subcutaneous tissues on the back of the mice. Consistent with peptide homing to BAT, dose-dependent PEP3-IRDye800 fluorescence was detected in the interscapular and perirenal areas for 30 and 60 nmol doses ( Fig. 5b ). Although signal was stronger shortly post-injection, it persisted after 24 h ( Fig. 5b ). Control peptide PEP1-IRDye800 localized to interscapular and perirenal areas at a significantly lower level ( Fig. 5b ). We also inspected fluorescence in isolated tissues better exposed for signal detection. Fluorescence was observed in BAT, but not in i.p. WAT, at a dose as low as 10 nmol of PEP3-IRDye800 per mouse and was dose-dependent ( Fig. 5c ). In contrast, the control PEP1-IRDye800 conjugate was undetectable in adipose tissues at this dose and displayed higher signal in i.p. WAT than in BAT at 30 nmol ( Fig. 5c ). 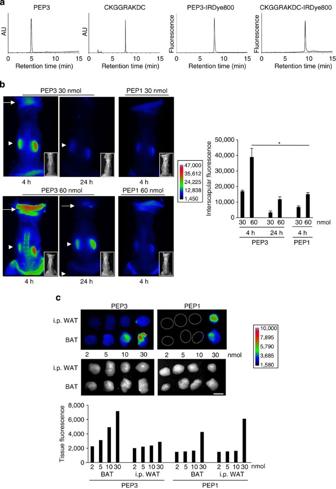Figure 5:Biodistribution of PEP3 conjugated with a NIR fluorophore. (a) HPLC chromatograms of peptide probes. Left: UV detection of PEP3 and WAT-homing peptide CKGGRAKDC (containing two Dde protecting groups on internal Lys residues) at 280 nm. AU denotes relative absorption units. Right: fluorescence detection of PEP3-IRDye800, and CKGGRAKDC-IRDye800. (b) Whole-body NIR-fluorescence imaging of cold-acclimated mice 4 and 24 h after i.v. administration of indicated doses of IRDye800-conjugated PEP3 or control PEP1. Arrows: interscapular signal; arrowheads: perirenal signal. Insets show black/white photographs of mice that had skin removed from the back for imaging. Right: plotted data analysis fromn=3 mice per group (mean ± s.e.m., *P<0.05, Student’st-test). (c) NIR-fluorescence imaging of i.p. WAT and interscapular BAT isolated from cold-acclimated mice i.v.-injected with increasing doses of IRDye800-conjugated PEP3 or a control peptide (PEP1) after 1 h of circulation. Scale shows fluorescence intensity. Black/white photographs of tissues are shown below. Scale bar, 5 mm. Graph: plotted quantitative data corresponding to NIR images. Figure 5: Biodistribution of PEP3 conjugated with a NIR fluorophore . ( a ) HPLC chromatograms of peptide probes. Left: UV detection of PEP3 and WAT-homing peptide CKGGRAKDC (containing two Dde protecting groups on internal Lys residues) at 280 nm. AU denotes relative absorption units. Right: fluorescence detection of PEP3-IRDye800, and CKGGRAKDC-IRDye800. ( b ) Whole-body NIR-fluorescence imaging of cold-acclimated mice 4 and 24 h after i.v. administration of indicated doses of IRDye800-conjugated PEP3 or control PEP1. Arrows: interscapular signal; arrowheads: perirenal signal. Insets show black/white photographs of mice that had skin removed from the back for imaging. Right: plotted data analysis from n =3 mice per group (mean ± s.e.m., * P <0.05, Student’s t -test). ( c ) NIR-fluorescence imaging of i.p. WAT and interscapular BAT isolated from cold-acclimated mice i.v.-injected with increasing doses of IRDye800-conjugated PEP3 or a control peptide (PEP1) after 1 h of circulation. Scale shows fluorescence intensity. Black/white photographs of tissues are shown below. Scale bar, 5 mm. Graph: plotted quantitative data corresponding to NIR images. Full size image To investigate how metabolic activity of BAT affects the tissue-homing capacity of PEP3-IRDye800, we performed a comparative analysis of its tissue distribution upon injection into warm- and cold-acclimated C57BL/6 mice. In addition, we used propranolol, a beta-adrenergic blocker [9] , to inhibit metabolic activity of tissues. Upon FDG injection, PET/CT imaging of the experimental animals demonstrated a 1.7-fold reduction in FDG uptake by BAT as a result of warm-acclimation; the reduction was 4.1-fold when warm-acclimation was combined with propranolol treatment ( Fig. 6a ). Injection of mice pre-conditioned in this manner with PEP3-IRDye800 and subsequent NIR-fluorescence imaging of resected tissues showed that BAT PEP3 signal was not significantly different in the cohorts analysed ( Fig. 6b ); signal was also detected in sc WAT for all cohorts. Consistent with the notion that i.p. WAT is less amenable to ‘browning’ than sc WAT [22] , only weak PEP3 signal was observed for i.p. WAT ( Fig. 6b ). In contrast to PEP3, the IRDye800-conjugated control peptide CKGGRAKDC displayed the expected accumulation in WAT, but not in BAT ( Fig. 6b ). 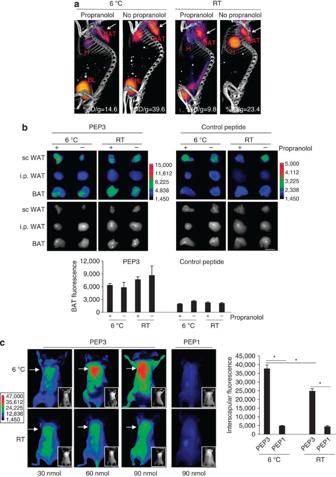Figure 6: Whole-body NIR-fluorescent imaging with a PEP3-directed probe. (a) Modulation of metabolism by warm-acclimation combined with propranolol treatment. Shown are PET/CT images of 6 °C- and RT-acclimated mice that were i.p. injected with propranolol where indicated. Note decreased FDG uptake by interscapular BAT (arrow) and heart (H) in propranolol-treated mice. FDG uptake in BAT is quantified as per cent injected dose per gram (%ID g−1). BL: bladder. (b) Tissues isolated from mice pre-conditioned as in (a) 1 h after i.v.-injection with 100 nmol of IRDye800-conjugates of PEP3 or a control WAT-homing peptide CKGGRAKDC18. NIR-fluorescent imaging demonstrates accumulation of PEP3 in interscapular BAT and sc WAT, but not in i.p. WAT in all groups, while CKGGRAKDC accumulates in WAT but not in BAT. Black/white photographs of tissue are shown below. Scale bar, 5 mm. Graph: Plotted data analysis fromn=3 mice per group (mean ± s.e.m.). (c) Whole-body NIR-fluorescence imaging of cold (6 °C) or warm (RT) -acclimated mice 1 h after i.v. administration of indicated doses of IRDye800-conjugated PEP3 or control PEP1. Arrow indicates interscapular area. Insets show black/white photographs of mice that were shaved for imaging (skin left on). Scale shows fluorescence intensity. Graph: plotted data analysis fromn=3 mice per group (mean±s.e.m., *P<0.05, Student’st-test). Figure 6: Whole-body NIR-fluorescent imaging with a PEP3-directed probe. ( a ) Modulation of metabolism by warm-acclimation combined with propranolol treatment. Shown are PET/CT images of 6 °C- and RT-acclimated mice that were i.p. injected with propranolol where indicated. Note decreased FDG uptake by interscapular BAT (arrow) and heart (H) in propranolol-treated mice. FDG uptake in BAT is quantified as per cent injected do s e per gram (%ID g −1 ). BL: bladder. ( b ) Tissues isolated from mice pre-conditioned as in ( a ) 1 h after i.v.-injection with 100 nmol of IRDye800-conjugates of PEP3 or a control WAT-homing peptide CKGGRAKDC [18] . NIR-fluorescent imaging demonstrates accumulation of PEP3 in interscapular BAT and sc WAT, but not in i.p. WAT in all groups, while CKGGRAKDC accumulates in WAT but not in BAT. Black/white photographs of tissue are shown below. Scale bar, 5 mm. Graph: Plotted data analysis from n =3 mice per group (mean ± s.e.m.). ( c ) Whole-body NIR-fluorescence imaging of cold (6 °C) or warm (RT) -acclimated mice 1 h after i.v. administration of indicated doses of IRDye800-conjugated PEP3 or control PEP1. Arrow indicates interscapular area. Insets show black/white photographs of mice that were shaved for imaging (skin left on). Scale shows fluorescence intensity. Graph: plotted data analysis from n =3 mice per group (mean±s.e.m., * P <0.05, Student’s t -test). Full size image Finally, we tested whether PEP3 could be used for non-invasive imaging of BAT. We injected increasing doses of IRDye800-conjugated peptides into mice pre-housed at 6 °C or RT and whole-body imaging was performed on animals that were shaved but had skin intact. Dose-dependent NIR interscapular fluorescence was detected at the dose of 30 nmol and higher for PEP3-IRDye800, while control PEP1-IRDye800 displayed significantly lower signal at matched concentrations ( Fig. 6c ). Consistent with PEP3 identified in isolated sc WAT ( Fig. 6b ), there was a diffuse signal throughout the torso. However, observation of the strongest signal in the interscapular area ( Fig. 6c ) indicates that peptide homing to BAT is detectable by non-invasive imaging. Higher interscapular signal in cold-acclimated mice ( P =0.01, Student’s t -test) suggests increased expression of PEP3 receptor in the vasculature of metabolically active BAT. In addition, increased interscapular signal in cold-acclimated mice could be partly explained by PEP3 homing to interscapular beige sc WAT metabolically activated upon cold acclimation. Previous studies had laid out the foundation for non-invasive methods to image BAT with fluorescent dyes [31] ; however, the lack of BAT-specific probes has limited their applicability. With the goal of establishing new approaches for BAT detection in the body, here we tested the capacity of peptides isolated from combinatorial libraries to serve as imaging probes. Combined, our data indicate that PEP3, a peptide binding to the endothelium, has selectivity for BAT and metabolically active beige adipose tissue found within sc WAT. Our data provide a proof of concept that BAT can be detected via ligand-directed fluorescent probe delivery. We demonstrate that PEP3 can be used to identify the major BAT depots by whole-body NIR-fluorescence imaging. Previously, we have used organ-homing peptides as ‘baits’ for isolation of the corresponding biological receptors [12] , [18] . Identification of the cell surface receptor for PEP3, which is beyond the scope of this study, might lead to the discovery of new molecular networks operating in the context of BAT vasculature, with implications for our understanding of adipose biology and for drug discovery. Localization of PEP3 to sc WAT, elevated in cold-acclimated animals, indicates that its receptor is expressed in the vasculature associated not only with BAT but also with beige adipose tissue. The revealed conservation of endothelial markers in the vasculature of BAT and sc WAT is not surprising in light of the recent studies indicating the common origin of BAT and of certain sc WAT depots [32] . Future studies will establish if the white/beige adipose tissue conversion [21] , [28] could be monitored with probes against PEP3 receptor. Although the probe characterized here reliably discriminates i.p. WAT from other types of adipose tissue, future efforts may identify new molecules enabling a more specific targeting of each individual type of adipose tissue found in the body. Each peptide in this study contains the chelation moiety 1,4,7-triazacyclononane, 1-glutaric acid-4,7 acetic acid (NODAGA), which can be used for dual labelling of fluorescent peptides with a radioisotope in future applications. The long-term objective of this study is to develop ligand-guided imaging probes for analysing BAT in humans. It remains to be tested whether PEP3 binds to a receptor expressed in human BAT vasculature. The currently practiced PET imaging can detect only metabolically active BAT and is prone to false-positive signals from other metabolically active tissues [9] , [10] . We show that PEP3 localizes to BAT endothelium without cold acclimation and UCP1 upregulation, and even upon metabolism blocking with propranolol. However, section analysis ( Fig. 4d ) and whole-body experiments ( Fig. 6c ) detected increased PEP3 accumulation in BAT of cold-stimulated animals, suggesting that metabolic activation increases PEP3 receptor bioavailability. As quantified in Fig. 4c,d , PEP3 also localizes to vasculature in browning areas of sc WAT, and its accumulation in both BAT and sc WAT increases upon sympathetic nervous system stimulation. Quantitative difference in PEP3 homing may be not fully reflected in Fig. 6b , because interscapular tissue analysis is prone to experimental error due to variability in the amount of resected BAT-associated WAT influencing the readout. Owing to the imprecision of whole-tissue imaging techniques used, it is currently not entirely clear to what extent BAT metabolic activity is a requisite for PEP3 homing. Despite the apparent limitations of PEP3, its discovery illustrates the potential of the screens for agents that may be useful as imaging probes homing to BAT without a need for its stimulation. Our work sets the foundation for future screens that may identify new probes useful for specific detection of individual BAT depots. The established approaches to perform peptide screens directly in humans [11] , [14] may expedite the progress in the field. Vascular-targeting peptide probes may also enable a way to monitor changes in highly dynamic body BAT/WAT distribution. Aging and obesity, resulting from excess accumulation of WAT, are associated with reduction in BAT [7] . Vice versa, obesity development may be restricted by the amount and/or activity of BAT [21] , [33] , which has opened new perspectives for obesity management [3] . Eventually, BAT probes optimized as a continuation of this study could also be used for the development of targeted vectors with the goal of stimulating residual BAT. This could, potentially, evolve into new obesity treatments based on shifting the balance in adipose tissue toward its conversion to metabolically active state. Animal experiments All animal studies were performed in accordance with the standards of the University of Texas Health Science Center-Houston (Houston, TX, USA) Department of Comparative Medicine after review and approval of the protocol by Institutional Animal Care and Use Committee /Animal Welfare Committee. Cold acclimation was performed for 1 week where indicated. The screen for BAT-homing peptides was performed in 6-week-old 129S6/SvEvTac (Sv129) males (Jackson) as described [12] , [13] , [18] by injecting 10 10 transforming units of the library into the tail vein and allowing the phage to circulate for 1 h. Recovered tissues were individually weighed, ground with a glass Dounce homogenizer, suspended in 1 ml of Dulbecco’s modified Eagle’s medium (DMEM) containing proteinase inhibitors (DMEM-prin), vortexed, and washed three times with DMEM-prin. Tissue homogenates were then incubated with 1 ml of host bacteria (log phase E. coli K91kan; OD 600 ~2). Aliquots of the bacterial culture were plated onto Luria–Bertani agar plates containing 40 μg ml −1 tetracycline and 100 μg ml −1 kanamycin. Plates were incubated overnight at 37 °C. In every selection round, phage recovered from BAT were amplified in K91 E. coli grown on plates and used for the next round. Peptide enrichment was assessed based on its recovery frequency among 96 phage peptide-coding inserts sequenced from PCR-amplified phage DNA [12] , [18] and clone accumulation in BAT and control tissues was quantified as the frequency of the sequence among all sequences analysed by using ClustlW software. Peptide homing validation studies were performed in 6-week-old C57BL/6 males (Jackson). Cell isolation and culture Organs were resected and cell suspensions were made as described [12] , [34] . Briefly, minced tissues was digested in 30 U ml −1 dispase (BD Biosciences) plus 0.5 mg ml −1 collagenase type I (Worthington Biochemical) solution under gentle agitation for 1 h at 37 °C, filtered on 70-μm Nitex filters, centrifuged at 200 g for 5 min to separate the stromal/vascular pellet from adipocytes, and extensively washed with PBS. Stromal/vascular cells adherent to uncoated plastic (overnight) in DMEM/fetal bovine serum (FBS) were washed with PBS to remove non-adherent cells. For white adipogenesis induction, cells grown to confluence were cultured in medium containing 1.7 mM insulin/0.5 mM IBMX, 1 mM dexamethasone/0.2 mM indomethacin for 3 days and 1.7 mM insulin afterwards [12] . For brown adipogenesis induction, medium containing 5 μM dexamethasone, 850 nM insulin, 1 nM T3 and 1 μM rosiglitazone was used [27] . Tissue section analysis Immunolocalization was performed in paraffin sections of 10% formalin-fixed tissues as described [12] . Briefly, upon deparaffinization in xylenes and ethanol, EDTA-based antigen retrieval was performed in a steamer for 30 min, followed by washing with 0.3% Triton X-100 and protein blocking in serum-free protein block (DAKO). Primary antibodies (4 °C, 12 h) and secondary antibodies (room temperature, 1 h) were applied to slides upon dilution with PBS containing 0.05% Tween 20. Primary antibodies used: rabbit anti-phage (Sigma-Aldrich, 1:300), goat anti-CD31 (Santa Cruz Biotechnology, 1:75), and rabbit anti-UCP1 (Abcam, 1:250). Secondary antibodies used: Alexa 488-conjugated (Invitrogen) and HRP-conjugated (DAKO). Biotinylated IB4 (Vector Labs, 1:50) was used with Alexa 488-conjugated streptavidin. Nuclei were stained with Hoechst 33258 or TOPRO3 (Invitrogen). Fluorescence images were acquired with an Olympus IX70 and Magnafire software (Olympus). Confocal images were acquired with TCS SP5/LAS AF software (Leica). For quantification, at least ten × 10 view fields per sample were analysed. Peptide accumulation in tissue was quantified by measuring cumulative pixel intensity in multiple fields of view by using Amira 5.4 (VSG) software. Flow cytometry For FACS, collagenase/dispase-digested interscapular BAT cells were pre-gated to exclude debris, cell clumps, contaminating polymorphonuclear cells, red blood cells, as well as dead cells based on 7-AAD staining and sorted into populations with FACSAria/FacsDiva software (BD Biosciences). Upon incubation with APC-anti-CD34 (RAM34), PE-anti-CD31 (MEC 13.3), and APC-Cy7-CD45 (30-F11) monoclonal IgG diluted according to the manufacturer’s recommendations (BD Biosciences), cells were gated first on CD31-CD45 cells and then on CD34+ cells. The corresponding isotype controls (BD Biosciences) and the positions of previously characterized hematopoietic and endothelial populations on the plots [12] , [26] were used to set gate cutoffs. Quantification of phage transforming unit recovered in host K91 E. coli resistant to tetracycline and kanamycin was performed as described above. Peptide synthesis and labelling Peptides were synthesized by Bachem (Torrance, CA) by stepwise Fmoc/tBu solid-phase peptide synthesis. A Lys residue and NODAGA-(tBu) 3 were sequentially added to the N-terminus of each peptide on solid phase. The synthesis was performed on a pre-loaded Fmoc-Ser(tBu)-Wang resin using DIC/HOBt activation and 20% piperidine (v/v) in DMF for Fmoc deprotection steps. At the conclusion of chain assembly, the completed peptide-resin was dried and global deprotection/cleavage performed using TFA:water:TIS (95: 2.5: 2.5) for 3 h at room temperature. Peptide CKGGRAKDC [18] was synthesized as above except it contained 1-(4,4-dimethyl-2,6-dioxocyclohex-1-ylidene)ethyl (Dde) protecting groups on the two internal Lys residues, which were not removed during global deprotection. The crude products were purified by high-performance liquid chromatography (HPLC) using a Vydac 218TP1022 preparative column and fractions above 90% purity (assayed by analytical HPLC, Fig. 5a ) were pooled and lyophilized. Cy3-conjugated PEP3 was generated using the EasyLink Cy3 Conjugation Kit (Abcam) by attaching Cy3 via the ε-amine of the N-terminal Lys residue. The crude product was HPLC-purified and characterized by electrospray ionization mass spectrometry (ESI-MS). ESI-MS (+) ( m/z ): calcd, 1871.2 (M+H); found, 1872.9 (M+H) + . Conjugation of IRDye800 (in the form of IRDye800CW NHS-ester) (LICOR Biosciences, Lincoln, NE) was performed by adding 2.5 mg (2.1 μmol) of dye to peptide solution (for PEP3: 2 mg, 1.4 μmol) in 0.1 M sodium phosphate buffer (pH 8.33) and reacting in the dark at RT for 4 h. The crude product was HPLC-purified (C-18 column: 5 μm, 9.4 × 250 mm 2 ) at 2 ml min −1 , with the mobile phase starting from 90% solvent A (0.1% TFA in water) and 10% solvent B (0.1% TFA in acetonitrile) to 10% solvent A and 90% solvent B for 20 min. The fraction containing the desired conjugate was collected, evaporated and stored in the dark at −20 °C. The pure conjugate was obtained in >82% yield. Analytical HPLC showed a major peak corresponding to the product at 7.7 min with >95% purity ( Fig. 5a ). ESI-MS (+) ( m/z ): calcd, 2410.6 (M+H); found, 1206.2 (M+2H) 2+ . IRDye800 conjugation to the CKGGRAKDC peptide was carried out in DMSO and underwent removal of the Dde protecting groups by stirring in DMF containing 2% hydrazine for 30 min at RT. The product was purified by HPLC to >95% ( Fig. 5a ) and analysed by ESI-MS. ESI-MS (+) ( m/z ): calcd, 2406.8 (M+H); found, 1204.3 (M+2H) 2+ . NIR imaging Experiments with three mice (6-week-old C57BL/6 males) per group were performed twice to ensure reproducibility. Mice were anaesthetized with 1% isoflurane. NIR-fluorescence images were acquired using a custom-built fluorescence imaging system [35] , [36] , [37] , [38] by illuminating a field of view with 785 nm of light from a 500-mW laser diode outfitted with a ‘clean up’ filter and expanded with a convex lens and diffuser to create a uniform excitation field. Emitted fluorescence at 830 nm was collected through two bandpass filters placed before a 28 mm Nikon camera lens. The images were captured by an electron-multiplying charge-coupled device camera (PhotonMax 512; Princeton Instruments, Princeton, NJ, USA) with 200–800 ms of integration time. For acquisition of white-light images, the optical filters were removed, and a low-power lamp illuminated the subject. Image acquisition was accomplished by V++ software (Auckland, New Zealand). In vivo small animal PET/CT imaging studies were performed using an Inveon dedicated PET docked with a multimodality CT (Siemens Medical Solutions, Knoxville, TN). The CT imaging parameters were an x-ray voltage of 80 kV with an anode current of 500 μA and an exposure time of 260 ms of each of the 120 rotation steps over the total rotation of 220° at low system magnification. After CT imaging, PET emission scans were performed 1 h after i.v. injection of FDG (7.4 MBq). PET and CT images were reconstructed using two-dimensional filtered back-projection and a Feldkamp cone-beam algorithm with a ramp filter cutoff at the Nyquist frequency, respectively. PET and CT image fusion and region-of-interest analysis were performed using the vendor software package to determine per cent injected dose/g (%ID g −1 ) values for each mouse. FDG uptake was blocked by propranolol (Sigma-Aldrich, St Louis, MO) administered i.p. at 5 mg kg −1 body weight 20 min before FDG and peptide injection. Statistical analysis Homoscedastic Student’s t -test was used, with P <0.05 considered significant. Validation experiments were repeated at least twice with similar results. How to cite this article: Azhdarinia, A. et al. A peptide probe for targeted brown adipose tissue imaging. Nat. Commun. 4:2472 doi: 10.1038/ncomms3472 (2013).